Dehydrated hereditary stomatocytosis linked to gain-of-function mutations in mechanically activated PIEZO1 ion channels Dehydrated hereditary stomatocytosis is a genetic condition with defective red blood cell membrane properties that causes an imbalance in intracellular cation concentrations. Recently, two missense mutations in the mechanically activated PIEZO1 ( FAM38A ) ion channel were associated with dehydrated hereditary stomatocytosis. However, it is not known how these mutations affect PIEZO1 function. Here, by combining linkage analysis and whole-exome sequencing in a large pedigree and Sanger sequencing in two additional kindreds and 11 unrelated dehydrated hereditary stomatocytosis cases, we identify three novel missense mutations and one recurrent duplication in PIEZO1 , demonstrating that it is the major gene for dehydrated hereditary stomatocytosis. All the dehydrated hereditary stomatocytosis-associated mutations locate at C-terminal half of PIEZO1. Remarkably, we find that all PIEZO1 mutations give rise to mechanically activated currents that inactivate more slowly than wild-type currents. This gain-of-function PIEZO1 phenotype provides insight that helps to explain the increased permeability of cations in red blood cells of dehydrated hereditary stomatocytosis patients. Our findings also suggest a new role for mechanotransduction in red blood cell biology and pathophysiology. Dehydrated hereditary stomatocytosis, (DHS, Xerocytosis, MIM no. 194380) is a dominantly inherited pleiotropic syndrome characterized by increased permeability of red blood cell (RBC) membranes to cations (for review see Delaunay [1] ). It is typically associated with silent-to-mild haemolysis, pseudohyperkalaemia (that is, loss of K + from red cells on storage at room temperature), and perinatal oedema [2] . A minor proportion of the red cells appear as stomatocytes on blood films. As is frequently observed in chronic haemolytic diseases, complications such as splenomegaly, resulting from increased red cell trapping in the spleen, and cholelithiasis, resulting from elevated bilirubin levels, may occur. For unknown reasons, the course of DHS is frequently associated with iron overload that may lead to hepatosiderosis [3] . Two genetic loci have been associated with DHS. Linkage to locus 16q23-qter was demonstrated in 1998 (ref. 4 ), which we further refined to a 11.5-cM interval based on information available on a large three-generation pedigree [5] , an interval confirmed in another large Canadian kindred [6] . Recently, two missense mutations at the FAM38A gene lying in this interval and encoding the PIEZO1 protein (M2225R and R2456H) were associated to DHS in two large North-American pedigrees [7] . A second locus for DHS was identified on chromosome 2q35q36 for at least one family [8] , [9] . Very recently the Iolascon’s group identified two heterozygous missense gain-of-function mutations at a single residue (R375) in the ABCB6 gene causing familial pseudohyperkalemia, a related disorder, in three multigenerational families [10] . ABCB6 is a porphyrin transporter present in erythrocytes membranes. Whether ABCB6 and PIEZO1 act through a shared pathway is unknown. PIEZOs are newly identified mechanically activated (MA) cation channels. These ion channels are proposed homotetramers, with each subunit encompassing 30–40 transmembrane domains. They are expressed in many cell types including human erythroid progenitor cells [7] , [11] , [12] . Some insights into the roles of PIEZO1 have been obtained recently by knockdown experiments in mammalian epithelial cells from the kidney and the lung, and in lung cancer cells [13] , [14] . In the context of kidney epithelial cells, PIEZO1 is proposed to act as a sensor of cell tension. McHugh et al. demonstrated that PIEZO1 inactivation promotes cell migration of normal lung epithelial cells, and leads to a switch towards β-integrin-independent amoeboid migration of small lung cancer cells. Evidence for PIEZO function in vivo is still limited. In Drosophila , Piezo is required for mechanical nociception [15] , and as mentioned above, two human PIEZO1 mutations are associated with DHS patients described by Zacharykanski et al. [7] However, the mechanism by which these mutations alter channel properties and in turn cause the observed phenotype is yet to be elucidated. Here, we identify three additional missense mutations and one recurrent duplication mutation in PIEZO1 of DHS patients. Functional characterization of recombinant PIEZO1 channels containing any one of these mutations indicates that they are all gain-of-function mutations that could cause a net increase in ion flux leading to DHS. Mutation detection Our genetic analysis had begun when the gene causing DHS was not yet known. We first performed a whole-exome sequencing analysis using two distant affected subjects of our large previously described pedigree [5] ( Fig. 1 ). Predicted functional coding and unique variants were found at five genes contained in the linkage interval ( Supplementary Table S1 and Supplementary Fig. S1 ). Only two missense variants were not shared by the unaffected subject, the CDT1 and FAM38A — PIEZO 1 genes. Although CDT1 (chromatin licensing and DNA replication factor 1) belongs to a family of DNA replication proteins and is essential for DNA replication, PIEZO1 appeared as a more attractive candidate because of its recent identification as MA ion channels involved in mammalian mechanotransduction [12] . 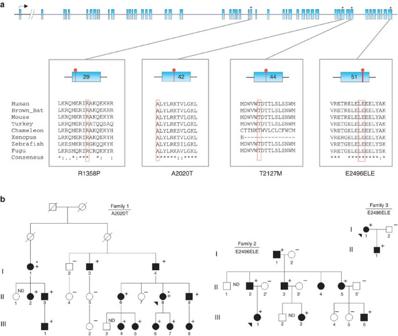Figure 1: Mutation screening results inPIEZO1among patients and relatives. (a) Graphical representation of the 51 exons of humanPIEZO1gene, with evolutionary proteic conservation analysis of the mutants surrounding regions amongst vertebrates. Blue boxes: exons. Red lollipops: location of the identified mutations. Red boxes in aligned sequences: amino-acid residues concerned by the mutations. (b) Pedigrees of the three French DHS families with corresponding mutations. Black arrowheads: index cases; asterisks: affected patients selected for exome sequencing;+ and −, respectively: presence or absence of the described mutation. Figure 1: Mutation screening results in PIEZO1 among patients and relatives. ( a ) Graphical representation of the 51 exons of human PIEZO1 gene, with evolutionary proteic conservation analysis of the mutants surrounding regions amongst vertebrates. Blue boxes: exons. Red lollipops: location of the identified mutations. Red boxes in aligned sequences: amino-acid residues concerned by the mutations. ( b ) Pedigrees of the three French DHS families with corresponding mutations. Black arrowheads: index cases; asterisks: affected patients selected for exome sequencing;+ and −, respectively: presence or absence of the described mutation. Full size image Genotyping of the PIEZO1 p.Ala2020Thr (A2020T) variant, identified by exome sequencing, in 14 affected and 5 unaffected members of the family 1 showed a complete co-segregation with the disease. Bioinformatic softwares (SIFT, Polyphen 2) showed a high likelihood of pathogenicity score ( Supplementary Table S2 ). We then performed a systematic screening of the entire coding sequence of PIEZO1 gene in a series of two other kindreds and 11 unrelated DHS cases. Index cases were referred to our centre for investigation of chronic Coombs test negative haemolysis, with few symptoms for most of them. DHS was diagnosed by ektacytometry, and showed the typical dehydrated profile in each case. As expected, the electrophoretic analysis of RBC membrane protein was normal. Other biological and clinical findings were in agreement with the DHS diagnosis ( Table 1 ). Three additional mutations were found in 10 subjects ( Table 1 ): two missense mutations, p.Arg1358Pro (R1358P) and p.Thr2127Met (T2127M), and a duplication of six nucleotides 5′-GGAGCT-3′ at the very end of exon 51, about 70 nucleotides before the stop codon ( Fig. 1 and Supplementary Fig. S2 ). This duplication (c. 7479_7484dup) occurs in a region of low complexity and rich in leucine (L) and glutamate (E) codons. The resulting staggered in-frame duplication of leucine 2,495 and glutamate 2,496 (p.Leu2495_Glu2496dup) will be addressed as E2496ELE. Table 1 Clinical and haematological presentation of the 11 index cases. Full size table We observed that E2496ELE was recurrently found in eight unrelated index cases ( Table 1 ). Haplotype analysis using single nucleotide polymorphisms (SNPs) at the PIEZO1 gene showed that this in-frame duplication was carried by at least four different haplotypes, thus excluding an ancestral allele ( Supplementary Table S3 ). A majority of available bioinformatic softwares could not predict its pathogenicity, but Mutation Taster considered it as possibly polymorphic. However, it was absent from the 1000 Genomes, Exome Variant Server, or dbSNP v135 databases. The four mutations were found in PIEZO1 motifs with a high level of conservation among vertebrates ( Fig. 1a ). We further assessed the frequency of E2496ELE in 600 healthy French controls and found it twice among 1,200 alleles (minor allele frequency (MAF)=0.0017), contrasting with a very highly significant proportion of mutated alleles in our DHS series (8/22, minor allele frequency=0.36, P <10 −76 ). Of note, one of the two positive healthy individuals was considered to have hyperkalaemia in one of his blood tests, with no additional information. Another argument for pathogenicity of this recurrent variant was provided by its co-segregation with DHS diagnosis in families 2 and 3 ( Fig. 1b ). In these two families, each positive subject had both pseudohyperkalaemia and abnormal haematologic parameters. The penetrance of the condition could therefore be considered as 100% in the tested individuals. 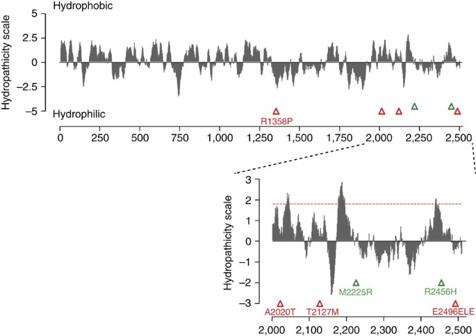Figure 2: Hydrophobicity plot of human PIEZO1 and position of reported mutations. Kyte-Doolittle hydrophobicity analysis (19 residues window) of human PIEZO1 prepared using the ProtScale program (Expasy). Triangles indicate the position of previously reported (green) and newly identified (red) mutations associated with DHS. Inset: magnification of C-terminal region. Peaks with scores greater than 1.8 (red dashed line) indicate possible transmembrane regions. No obvious/simple genotype–phenotype relationship appear from our data; however, we noticed that this restricted sample of eight index cases bearing the E2496ELE mutation had a tendency for lower age at diagnosis (20.5 versus 60.6 years) and a more severe haematological phenotype compared to the three index cases carrying a missense mutation ( Table 2 ). This observation needs to be confirmed with larger number of subjects. Overall, four different mutations lying in highly conserved C-terminal regions of the PIEZO1 protein ( Fig. 2 ) were found in 11 unrelated familial and sporadic DHS cases with strong arguments of pathogenicity for each of them. Table 2 Clinical and haematological comparison between index patients with PIEZO1 mutations. Full size table Figure 2: Hydrophobicity plot of human PIEZO1 and position of reported mutations. Kyte-Doolittle hydrophobicity analysis (19 residues window) of human PIEZO1 prepared using the ProtScale program (Expasy). Triangles indicate the position of previously reported (green) and newly identified (red) mutations associated with DHS. Inset: magnification of C-terminal region. Peaks with scores greater than 1.8 (red dashed line) indicate possible transmembrane regions. Full size image Electrophysiological studies of DHS mutations in hPIEZO1 channels We then set out to determine whether these mutations alter PIEZO1 channel activity. We introduced the four mutations identified from our study (R1358P, A2020T, T2127M and E2496ELE) and the two previously published (M2225R and R2456H) DHS-associated mutations [7] in hPIEZO1 full-length complementary DNA. We transfected HEK293T cells with wild-type (WT) or mutant hPIEZO1 and analysed channel activity via whole-cell patch clamp configuration. MA inward currents were recorded by applying mechanical force on to the cell surface using a glass probe [12] ( Fig. 3a ). In cells expressing WT hPIEZO1 such stimulation gives rise to rapid transient increase in current. 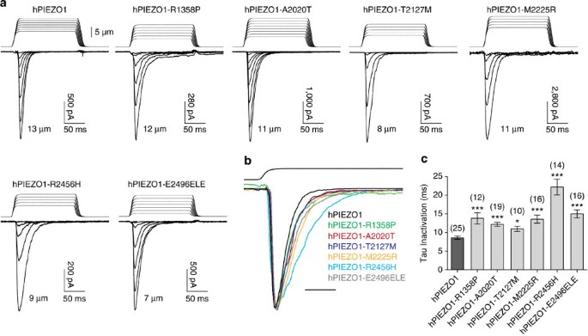Figure 3: Recombinant hPIEZO1 channels with DHS-associated mutations display slow inactivation kinetics. (a) Representative traces of mechanically activated inward currents recorded at −80 mV from HEK293T cells expressing either WT or indicated mutant hPIEZO1. Cells were stimulated by a series of mechanical steps (150 ms duration) in 1 μm increments. For each representative trace, the channel response corresponds to the indentation distance of the glass probe and is shown as a series of responses starting from the step that generates the first mechanically activated current (the initial steps that did not cause channel activation are not shown) till the step that generates the maximum response for that cell. The distance of the probe for the maximum response for each construct is indicated. (b) Representative WT (black) and mutant (coloured) hPIEZO1 traces normalized to peak. Maximum currents from each construct shown inaare overlaid to highlight difference in inactivation kinetics. Scale bar; 25 ms. (c) Average of inactivation time constant (tau, ms) for WT and mutant hPIEZO1 channels. Bars represent mean±s.e.m. and numbers in parenthesis indicate number of cells tested for each condition. *P<0.05, ***P<0.001; relative to WT hPIEZO1 (Student’st-test). Figure 3: Recombinant hPIEZO1 channels with DHS-associated mutations display slow inactivation kinetics. ( a ) Representative traces of mechanically activated inward currents recorded at −80 mV from HEK293T cells expressing either WT or indicated mutant hPIEZO1. Cells were stimulated by a series of mechanical steps (150 ms duration) in 1 μm increments. For each representative trace, the channel response corresponds to the indentation distance of the glass probe and is shown as a series of responses starting from the step that generates the first mechanically activated current (the initial steps that did not cause channel activation are not shown) till the step that generates the maximum response for that cell. The distance of the probe for the maximum response for each construct is indicated. ( b ) Representative WT (black) and mutant (coloured) hPIEZO1 traces normalized to peak. Maximum currents from each construct shown in a are overlaid to highlight difference in inactivation kinetics. Scale bar; 25 ms. ( c ) Average of inactivation time constant (tau, ms) for WT and mutant hPIEZO1 channels. Bars represent mean±s.e.m. and numbers in parenthesis indicate number of cells tested for each condition. * P <0.05, *** P <0.001; relative to WT hPIEZO1 (Student’s t -test). Full size image Sensitivity of a channel to mechanical stimulation, which can also be expressed as the distance of the mechanical stimulus, can be estimated by measuring ‘threshold’ values for each cell. We measure this by subtracting the distance at which the probe first touches the cell surface from the minimal distance at which MA currents are evoked. Threshold is therefore merely the distance of indentation, after making cell contact, required to activate the channel. We observed no apparent differences in threshold values for any of the hPIEZO1 mutants relative to WT hPIEZO1, suggesting that the DHS mutations do not alter the channel’s sensitivity to mechanical stimulation ( Table 3 ). Table 3 Inactivation kinetics of hPIEZO1 mutations. Full size table Similar to WT hPIEZO1, all the mutants had a linear current–voltage correlation with a reversal potential close to 0 mV ( Supplementary Fig. S3 ). At −80 mV, the maximum current ( I max ) recorded from cells expressing mutant hPIEZO1 channels was found to be similar to that of WT hPIEZO1 ( Table 3 ). A potential exception to this was M2225R-induced currents, which showed overall larger I max currents. However, the average was not significantly different compared with WT. In addition, peak currents depend on expression levels in HEK293T cells, and might not represent endogenous expression. All WT and mutant hPIEZO1 MA inactivation currents could be fit with a mono-exponential function. Remarkably, we observed that all mutations caused considerable increase in the inactivation time constant relative to WT channel kinetics ( Fig. 3b ). The R2456H mutation had the maximum impact with a 2.6-fold slower time constant, while the remaining five mutations inactivate with 1.3- to 1.7-fold slower kinetics ( Fig. 3c and Table 3 ). Therefore, all six mutations can be defined as gain-of-function, as they would give rise to an increased channel activity in response to a given mechanical stimulus. We present a comprehensive analysis of DHS-causing PIEZO1 mutations. Four novel PIEZO1 mutations were identified in 11 out of 14 index cases, demonstrating that this gene has a major role in DHS. DHS is a difficult diagnosis because of a highly variable clinical expression, ranging from the absence of clinical symptoms to lethal perinatal oedema. Other features of DHS include severe iron overload leading to hepatic transplantation, or life-threatening thromboembolic disease after splenectomy. But the most frequent DHS condition is moderately symptomatic haemolysis. The only biological test for DHS is ektacytometry, which is available in a very limited number of laboratories. The disease may be overlooked for years or decades and is sometimes confused with spherocytosis. Our data, including the presence of a recurrent mutation, render a genetic diagnosis possible. PIEZO1 is a large homotetrameric mechanosensitive ion channel with each subunit containing 2,521 amino acids and predicted to encompass no less than 30 transmembrane domains [11] . However, PIEZOs do not share homology with any known ion channels or proteins. Interestingly, all six DHS-associated PIEZO1 mutations are located in the second half of the coding sequence. Indeed, apart from R1358P, all are in the C terminal 1/5th of the protein, albeit distributed across several exons in the gene. It is difficult to conclude too much from this information, as we know virtually nothing about the topology of PIEZO1, or the role of different PIEZO regions in channel function. However, our electrophysiological studies implicate the C-terminal region in regulating gating kinetics. Human PIEZO1 is a very polymorphic gene. As an example, many coding variants of PIEZO1 are present in the 1,000 genomes database, including variants predicted as deleterious. Interestingly, the distribution of these variants tends to cluster to the N- terminal end of the protein, unlike DHS mutations ( Supplementary Fig. S1 ), suggesting an increasing selective pressure from the N terminal to the C-terminal end of the protein. One surprising finding is the recurrence of the E2496ELE mutation, observed in 8 out of the 11 DHS PIEZO1-related cases. It was also found twice in 1,200 healthy controls of French origin. We had no access to the medical record of these two a priori asymptomatic subjects, but one of these two heterozygous carriers had hyperkalaemia. As mentioned above, this in-frame insertion can neither be explained by a founder effect nor could be considered as a polymorphism taking into account its rarity in the general population, its associated clear phenotype and its electrophysiological consequences. The six-nucleotide-inserted sequence ‘GGAGCT’ represents a short intragenic in-frame insertion, embedded in a low complexity surrounding sequence between positions 2,491 and 2,499. Slippage mutagenesis, leading to the addition or removal of one copy of a short tandem repeat, is probably responsible for this recurrence. In the human genome, microdeletions and microinsertions of >1 to <20 nt were found to be strongly associated with surrounding short tandem repeats, similar to the sequence surrounding this duplication [16] . Characterization of kinetic properties of mutant PIEZO1 channels showed a striking effect: all six DHS-causing mutations resulted in a similar slowing of inactivation kinetics. We propose that these mutations could affect the inactivation mechanism by either destabilizing the inactivated state or stabilize the channel in the open state thereby biasing the open to inactivated state equilibrium towards open, resulting in an increased Na + and Ca 2+ ion influx. RBCs are unique in that they circulate in the vascular system for 120 days and undergo constant mechanical stress, specifically through the capillaries and splenic cords. Stabilization of the open conformation of PIEZO1 channels in RBCs could also alter the transition between closed and open states of the channel leading to higher open probability compared with WT channels. This shift in kinetics could potentially also cause a slight increase in basal channel activity (independent of mechanical stimulation), which may also contribute to the DHS phenotype. Detailed kinetic analysis of these channels in the future should tell us more about the gating mechanism and how these mutations in PIEZO1 could lead to erythroid dysfunction. Our analysis here was restricted to heterologously expressed PIEZO1 mutants. Recording of MA currents from control and affected RBCs in the future could more directly link PIEZO1-dependent current characteristics and pathophysiology of DHS. It is possible that increased PIEZO1 activity could directly contribute to RBC dehydration observed in DHS patients. Human RBCs have a resting membrane potential of about −10 mV, and one possibility is that the gain-of-function mutations cause increase in influx of Na + and efflux of K + through PIEZO1 channels. Indirect mechanisms could also account for this phenotype. For example, PIEZO1-mediated rise in intracellular Ca 2+ concentration could induce K + efflux by the activation of Ca 2+ -activated K + channels, the Gardos channel. Gardos channels have been shown to have a vital role in physiological and pathological states of erythrocytes. Additionally, it has been shown that Gardos channel activation causes a reduction in erythrocyte cell volume [17] , [18] . Multiple cell types along with erythroid progenitor cells express PIEZO1 (ref. 7 ). The specific haematologic phenotype of DHS patients due to gain-of-function PIEZO1 mutants is therefore surprising. It is, however, important to note that DHS is a mostly tolerated disorder, and even the RBC phenotype is relatively subtle–as reflected by the modest changes of RBC constants such as mean cell volume and mean cell haemoglobin concentration or the weak (5–15%) number of stomatocytes [1] , [19] . Therefore, variations in minor modulating factors could impact which cell types show phenotypes in DHS patients. For example, RBCs might be more sensitive to increased cation flux compared with other cell types, or PIEZO1 channels expressed in RBCs might be modulated in a way that amplifies the consequences of the PIEZO1 mutations. Another intriguing possibility is that RBC plasma membranes experience more mechanical stress compared with other cells because of their unique membrane properties and constant movement during blood circulation. It is also possible that other cell types and tissues are affected in DHS patients, but these have remained unknown or unexplained because of these modulating factors and the possible subtleness of phenotype. Perinatal oedema that is inconstantly observed in DHS patients is such an example. PIEZO1 is expressed in endothelial cells (unpublished data) and this phenotype could be the consequence of a leak out of the vascular compartment at a specific development stage. PIEZO1 has been implicated in cell–cell and cell–matrix interactions [20] . In both PIEZO1 knockdown experiments [13] , [14] , the mechanosensitivity and gating properties of the protein were not assessed, but the influence of PIEZO1 on cell migration/invasion and extrusion was described. The function of a mechanosensitive PIEZO1 channel in normal RBCs remains speculative. Erythrocytes are highly deformable cells, a property that allows them to pass though narrow capillaries of the microvasculature [21] . Mechanosensory feedback mechanisms could allow the cell to respond to its changing mechanical environment, possibly by regulating its volume and morphology. In this respect, it is interesting to comment on overhydrated hereditary stomatocytosis, another genetic disease that like DHS is associated with an imbalance in erythrocyte cation gradients. This disease is associated with mutations in Rhesus-associated glycoprotein, and is characterized by a dramatic reduction of stomatin from erythrocyte membranes [1] , [22] , [23] . Strikingly, stomatin family members from mouse and worm have been shown to be required for mechanotransduction in sensory neurons [24] , [25] , [26] . This tantalizing coincidence raises the possibility that the various genetic conditions that cause stomatocytosis are caused by disrupted mechanotransduction, and that perhaps PIEZOs and stomatin family members function in the same pathway. Yet another clue towards a role for mechanotransduction in erythrocytes comes from sickle cell disease, arguably the best-known erythrocyte disorder. In sickle RBCs, mutant haemoglobin molecules form large polymers under low oxygen conditions, which cause the deformation of the erythrocyte. This deformation coincides with the development of a cationic membrane current, termed pSickle, and subsequent erythrocyte dehydration [17] . Notably pSickle is blocked by a blocker of stretch-activated currents, the tarantula toxin Gsmtx4, which is also known to block PIEZO1 (refs 27 – 29 ). Future studies will explore the relationship between PIEZO1 and pSickle. In conclusion, we identify four new PIEZO1 mutations in DHS patients, demonstrating that PIEZO1 is a major determinant of DHS. We also present the first functional analysis of DHS-causing PIEZO1 mutations. Our studies provide a substantial step towards understanding physiopathology of DHS. Our findings will also be useful to establish DHS genotype/phenotype relationship and to refine the classification of RBC cation leak disorders on a molecular basis. During the final revision of this manuscript, two related papers were published which also show that DHS mutations in PIEZO1 alter channel activity [30] , [31] . Patients Our study focused on three families and 11 independent index cases with a typical DHS clinical and biological phenotype. Patients were from all regions of France, and were diagnosed through specialized consultation by a haematologist or a clinical geneticist. Some of the patients have been published elsewhere: family 1, which was described by us and others (family VA in Grootenboer et al. [2] and Beaurain et al. [5] , presented with mild, uncomplicated haematological signs of the disease, pseudohyperkalaemia and no history of perinatal oedema. In family 2 (family VE in Grootenboer et al. ) patients were affected by a mild-to-moderate haemolysis and anaemia, by a recurrence of perinatal oedema (three affected cases), and varying recurrence of pseudohyperkalaemia. Case 4 (ref. 3 ) and family 3 (refs 32 , 33 ) were case reports, these patients expressed a moderate form of anaemia and haemolysis without initial evidence of perinatal oedema or pseudohyperkalaemia. In these last three cases, diagnosis of DHS was done late after the onset of haematologic manifestations. The other cases were referred to the Haematology Department of the Hospital Kremlin-Bicêtre and their characteristics are summarized in Table 1 . Informed consents for genetic analysis were obtained for all patients, according to local institutional ethical board, Hôpital Européen Georges Pompidou Ethical Comitee. The research was conducted in the Hôpital Européen Georges Pompidou Genetics Department or the Haematology Department of Kremlin-Bicêtre University Hospital in Paris, France, and the Scripps Research Institute in San Diego, California. Haematological tests Blood electrolytes were measured in each center. RBC studies were performed in the same laboratory: cell counts and red cell constants were measured using an ADVIA 2120 (Siemens) instrument, blood smears were observed after May-Grünwald-Giemsa staining using standard methods, red cells membrane properties were assessed using osmolar gradient (ranging from 80 to 500 mosmol kg −1 ) ektacytometry using a Technicon ektacytometer and erythrocyte membrane proteins analysed by SDS–polyacrylamide gel electrophoresis as previously described [1] , [34] , [35] . Molecular genetics analysis and targeted exome sequencing Genomic DNA was extracted from EDTA blood samples using the QIAamp Midi Kit blood DNA extraction kit (Quiagen). Quality of the DNA was evaluated using nanodrop 2000 spectrophotometer (Thermo Scientific). Library preparation, capture, sequencing, and variants detection and annotation were performed by IntegraGen, Evry, France. Exons of genomic DNA samples were captured using Agilent in-solution enrichment methodology with their biotinylated oligonucleotides probes library, followed by paired-end 75 bp massively parallel sequencing on Illumina HiSeq 2000. For detailed explanations of the process, see Gnirke et al. [36] publication in Nature Biotechnology . Sequence capture, enrichment and elution were performed according to the manufacturer’s instruction and protocols (Human All exon kit V3, 50Mb, Agilent) without modification. Briefly, 3 μg of each genomic DNA were fragmented by sonication and purified to yield fragments of 150–200 bp. Paired-end adaptor oligonucleotides from Illumina were ligated on repaired A-tailed fragments, then purified and enriched by six PCR cycles. Six hundred nanograms of these purified libraries were hybridized to the SureSelect oligo probe capture library during 72 h. After hybridization, washing and elution, the eluted fraction was PCR amplified with 11 cycles, purified and quantified by qPCR to obtain sufficient DNA template for downstream applications. Each eluted-enriched DNA sample was then sequenced on an Illumina HiSeq 2000 as paired-end 75b reads. Image analysis and base calling were performed using Illumina Real Time Analysis Pipeline version 1.14 with default parameters. Bioinformatics analysis of PIEZO1 for exome study The bioinformatics analysis of deep sequencing data was based on the Illumina pipeline (CASAVA 1.8). CASAVA performs alignment of the reads to the human reference genome (hg19) with the alignment algorithm ELANDv2 (performs multiseed and gapped alignments), then calls the SNPs based on the allele calls and read depth, and detects variants (SNPs and Indels). Only the positions included in the bait coordinates were conserved. Genetic variations annotation was performed using IntegraGen in-house pipeline, which consists in gene annotation (RefSeq), detection of known polymorphisms (dbSNP v132, 1,000 genomes) followed by a mutation characterization (exonic, intronic, silent, nonsense and so on). For each position, the exomic frequencies (homo- and heterozygous) were determined from the IntegraGen Exome database, and the exome results provided by HapMap. Results were provided per sample and family upon tabulated text files, including coverage/depth statistical analysis per exome and per target. Genomic sequences of all 51 exons of PIEZO1 gene were amplified by PCR using either Red’y star reaction mix (Eurogentec) or Jumpstart reaction mix (Sigma). Twenty different primer pairs amplifying one or more exons each, targeting the unique reference transcript sequence of the gene (NM_001142864.2) were used. Sequencing reactions of the PCR products were performed using the Big Dye Terminator sequencing kit v3.3 (Life Technologies, Carlsbad, California, USA). Twenty-five additional primers were used to obtain the complete coding sequence of the gene from both strands. Sequencing products were migrated on an ABI prism 3730 sequencer (Life Technologies, Carlsbad, California, USA) and analysed using the Sequencher 5.0 software (Genecodes, Ann Arbor, Michigan, USA). Sequencing of PIEZO exon 51, for population frequency estimation of E2496ELE, was performed in 1,200 control alleles from a French healthy controls cohort. Primer pairs and PCR conditions are available upon request. Sequence alignment and analysis were performed using Sequencher software 5.0 (Genecodes, Ann Arbor, Michigan, USA). Sequence variations were analysed using Alamut (Interactive Biosoftware, Rouen, France), and predicted pathogenicity of variants was assessed using Polyphen 2, SIFT and Mutation Taster online tools. Frequency of variants in published populations were assessed in 1,000 genomes, Exome Variant Server and dbSNP databases. Human to other vertebrates protein alignments of PIEZO1 were performed using CLUSTAL Omega. All web tools addresses are listed in the Supplementary Table S4 . Cloning and tissue culture Halo-tagged hPIEZO1 was purchased from Kazusa DNA Research Institute. This clone differs from the NCBI sequence with coding differences at I83T, V250A, V394L and R407G and non-coding differences at codons 1338, 1846, 2190, 2214 and 2353. We first confirmed the functionality of the clone through electrophysiological experiments. The cDNA was then cloned into pIRES2–eGFP expression vector, and the DHS mutations were generated either by overlapping PCR mutagenesis or by using Agilent’s QuikChange II XL Site Directed Mutagenesis Kit (Stratagene) according to the manufacturer’s instructions. All clones were verified by full-length DNA sequencing. Human embryonic kidney 293T (HEK293T) cells were grown in DMEM containing 4.5 mg ml −1 glucose, 10% fetal bovine serum, 50 U ml −1 penicillin and 50 mg ml −1 streptomycin. Cells were plated onto poly-lysine-coated 12-mm round glass coverslips placed in 24-well plates and transfected using lipofectamine 2000 (Invitrogen) according to the manufacturer’s instruction. Plasmid DNA (600 ng ml −1 )was transfected and green fluorescent protein-positive cells were recorded from, 12–48 h post transfection. Electrophysiology and mechanical stimulation Patch clamp experiments were performed in standard whole-cell recordings using an Axopatch 200B amplifier (Axon Instruments). Patch pipettes had a resistance of 1.5–3 MΩ when filled with intracellular solution consisting of (in mM) 133 CsCl, 5 EGTA, 1 CaCl 2 , 1 MgCl 2 , 10 HEPES, 4 MgATP and 0.4 Na 2 GTP (pH adjusted to 7.3 with CsOH). The extracellular solution consisted of (in mM) 130 NaCl, 3 KCl, 1 MgCl 2 , 2.5 CaCl 2 , 10 HEPES and 10 glucose (pH adjusted to 7.3 with NaOH). All experiments were done at room temperature. Currents were sampled at 20 kHz and filtered at 2 kHz. Voltages were not corrected for a liquid junction potential. Leak currents before mechanical stimulations were subtracted off-line from the current traces. Mechanical stimulation was achieved using a fire-polished glass pipette (tip diameter 3–4 μm) positioned at an angle of 80° to the recording cell. Downward movement of the probe towards the cell was driven by a Clampex controlled piezo-electric crystal microstage (E625 LVPZT Controller/Amplifier; Physik Instrumente). The probe had a velocity of 1 μm ms −1 during the ramp segment of the command for forward motion and the stimulus was applied for 150 ms. To assess the mechanical sensitivity of a cell, the probe is first placed as close to the cell as possible (this distance could vary from cell to cell). Then, a series of mechanical steps in 1-μm increments was applied every 10 s, which allowed full recovery of mechanosensitive currents. Threshold was calculated by subtracting the distance at which the probe first touches the cell surface from the minimal distance at which MA currents are evoked. MA inward currents were recorded at a holding potential of −80 mV. For I–V relationship recordings, voltage steps were applied 0.7 s before the mechanical stimulation from a holding potential of −60 mV. Statistical analysis Frequency comparisons of variants were done using Fisher exact test. Clinical and haematological quantitative variables comparisons between subsets of patients were done using Student’s t -tests. Channel kinetic properties between WT and mutant PIEZO1 were compared using Student’s t -test. How to cite this article: Albuisson, J. et al. Dehydrated Hereditary stomatocytosis linked to gain-of-function mutations in mechanically activated PIEZO1 ion channels. Nat. Commun. 4:1884 doi: 10.1038/ncomms2899 (2013).